In vivoimaging of specific drug–target binding at subcellular resolution The possibility of measuring binding of small-molecule drugs to desired targets in live cells could provide a better understanding of drug action. However, current approaches mostly yield static data, require lysis or rely on indirect assays and thus often provide an incomplete understanding of drug action. Here, we present a multiphoton fluorescence anisotropy microscopy live cell imaging technique to measure and map drug–target interaction in real time at subcellular resolution. This approach is generally applicable using any fluorescently labelled drug and enables high-resolution spatial and temporal mapping of bound and unbound drug distribution. To illustrate our approach we measure intracellular target engagement of the chemotherapeutic Olaparib, a poly(ADP-ribose) polymerase inhibitor, in live cells and within a tumour in vivo . These results are the first generalizable approach to directly measure drug–target binding in vivo and present a promising tool to enhance understanding of drug activity. Small-molecule therapeutic drugs typically exert their effects through binding to one or a few protein targets. This critical interaction—a prerequisite of therapeutic drug efficacy—is often poorly understood and can generally not be visualized in live cells or entire organisms due to the lack of methods to directly measure drug–target engagement in a biological setting. As a result, most of our knowledge is incomplete, as it relies on target extraction assay systems [1] , [2] or indirect measurements where critical spatiotemporal information is lost, which further complicates drug development [3] . Recent advances in chemical techniques have allowed the creation of fluorescent drugs, prodrugs and activity-based probes to interrogate target engagement [4] , [5] , [6] . To date, most of these compounds have been used in vitro while a select few have been used in vivo for imaging drug distribution (pharmacokinetics) [7] or tumour detection [8] . However, to realize the full potential of intravital imaging with fluorescently labelled compounds determination of target engagement with subcellular resolution is needed [2] , [9] . We hypothesized that fluorescence polarization (FP) could be used to accurately measure drug binding in vitro and in vivo through multiphoton microscopy. FP [10] quantifies the degree of fluorescence depolarization with respect to the polarization excitation plane, providing insight into the state or environment of the excited fluorescent molecule. FP has been extensively used in non-imaging, plate reader and kinetic in vitro assays to measure numerous fluorescent molecule and molecular drug interactions including target engagement [11] , [12] . Extending FP to optical microscopy imaging modalities could provide spatially and temporally resolved mapping, enabling live cell imaging of target engagement of small-molecule drugs. However, microscopy imaging methods based on FP [13] have been more commonly used to study homo-FRET in membrane dynamics [14] , [15] , [16] , structure in ordered biological systems [17] , [18] and endogenous small molecules [19] or labelled protein interactions [20] . Herein we present multiphoton fluorescence anisotropy microscopy (MFAM) to image intracellular drug–target binding distribution in vivo . Specifically we demonstrate, with a Phase III drug candidate, that our approach is not only applicable to live cultured cells but also enables real-time imaging of drug–target engagement in vivo with submicron resolution. Fluorescence anisotropy and imaging set-up characterization Following photoselection under polarized excitation, all excited fluorophores are aligned with the same emission dipole orientation. However, due to the presence of rotational Brownian motion, fluorophores rotate with a correlation time ( τ θ ) dependent on viscosity, molecule size and temperature [21] . If the excited fluorophore is free to rapidly rotate on a timescale that is shorter than its fluorescence lifetime ( τ θ << τ ), emission will be isotropic (depolarized). However, when rotating slowly, the rotational correlation time will increase ( τ θ >> τ ) and emission will be preferentially aligned along one axis ( Fig. 1a ). Furthermore, a change in the fluorescence lifetime will also affect the emission polarization as molecules will have less or more time to rotate before emission. To characterize the extent of linearly polarized emission, fluorescence anisotropy (FA), a dimensionless parameter similar to FP and independent of excitation intensity ( Supplementary Fig. 1 , Supplementary Methods ), can be calculated. Thus, measurements of anisotropy provide insight into the rotational diffusion rate of molecules, which can be used in term to directly determine drug engagement with the target. 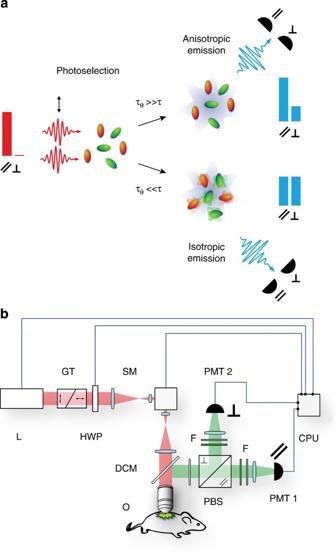Figure 1: Imaging set-up. (a) Schematic representation of the two-photon photoselection process in a randomly oriented distribution of fluorophores and the resulting fluorescence emission for low (isotropic) and high (anisotropic) rotational correlation times (τθ). Blue bars indicate schematically the distribution of emission along the two orthogonal linear polarization components (||,⊥) as measured at the two detectors, for the two cases. Orange particles represent excited molecules. (b) The optical set-up of the MFAM is based on a custom-modified Olympus FV1000-MPE (Olympus, USA) laser scanning microscopy system equipped with an upright BX61-WI microscope (Olympus, USA). Excitation light (red beam) from a Ti:sapphire laser (L) is filtered to select a linear state of polarization and then focused onto the imaged sample. Emitted fluorescent light (green beam) is epi-collected, separated into two linearly polarized orthogonal components and spectrally filtered before non-descanned detection. GT, Glan–Thompson polarizer; HWP, half-wave plate; SM, scanning mirrors; DCM, dichroic mirror; O, objective; PBS, polarization beam splitter; F, band-pass filters; PMT, photomultiplier tube; CPU, computer. Figure 1: Imaging set-up. ( a ) Schematic representation of the two-photon photoselection process in a randomly oriented distribution of fluorophores and the resulting fluorescence emission for low (isotropic) and high (anisotropic) rotational correlation times ( τ θ ). Blue bars indicate schematically the distribution of emission along the two orthogonal linear polarization components (||, ⊥ ) as measured at the two detectors, for the two cases. Orange particles represent excited molecules. ( b ) The optical set-up of the MFAM is based on a custom-modified Olympus FV1000-MPE (Olympus, USA) laser scanning microscopy system equipped with an upright BX61-WI microscope (Olympus, USA). Excitation light (red beam) from a Ti:sapphire laser (L) is filtered to select a linear state of polarization and then focused onto the imaged sample. Emitted fluorescent light (green beam) is epi-collected, separated into two linearly polarized orthogonal components and spectrally filtered before non-descanned detection. GT, Glan–Thompson polarizer; HWP, half-wave plate; SM, scanning mirrors; DCM, dichroic mirror; O, objective; PBS, polarization beam splitter; F, band-pass filters; PMT, photomultiplier tube; CPU, computer. Full size image Using multiphoton microscopy for anisotropy [22] offers several advantages over other imaging modalities. Extended light penetration depth enables relatively deep imaging in tissues in a physiologically relevant context, while a diminished scattering component in the near infrared reduces tissue scattering [23] . Therefore, multiphoton microscopy, with its low phototoxicity and high axial resolution, is ideally suited for high-resolution drug–target interaction imaging within single cells. MFAM imaging was developed using a custom-adapted commercial unit ( Fig. 1b ). We first tested the imaging system by measuring the viscosity dependence of anisotropy for pentamethyl–BODIPY (Me 5 –BODIPY), an ideal fluorophore for FA ( Supplementary Methods ), in increasing concentration of aqueous glycerol ( Fig. 2 and Supplementary Fig. 2 ). As expected, the measured anisotropy increased with increasing viscosity. The superior photoselectivity by two-photon excitation compared with single-photon absorption [24] significantly increased anisotropy values through enhanced photoselection, resulting in increased sensitivity ( Supplementary Fig. 3 ). Although high numerical aperture objectives are well known to produce distorted anisotropy values at the periphery of an image [25] (with small impact on-axis), restricting the field of view eliminates these aberrations ( Supplementary Figs 4 and 5 , Supplementary Methods ). 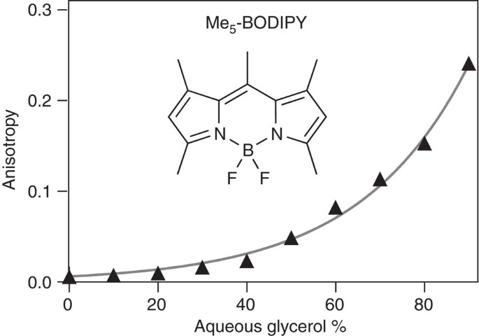Figure 2: Anisotropy measurement. Me5–BODIPY anisotropy dependence on viscosity, as measured in glycerol with MFAM. Measurements are obtained from two-photon images of sample drops of Me5–BODIPY and calculating the anisotropy of each pixel. Average±s.d. (n=6), fitted curve added for trend visualization. Figure 2: Anisotropy measurement. Me 5 –BODIPY anisotropy dependence on viscosity, as measured in glycerol with MFAM. Measurements are obtained from two-photon images of sample drops of Me 5 –BODIPY and calculating the anisotropy of each pixel. Average±s.d. ( n =6), fitted curve added for trend visualization. Full size image The resolution of the imaging system was determined using fluorescent microspheres. Both planar and axial measurements of a microsphere point spread function ( Fig. 3a ) demonstrate the high optical resolution of FA, making MFAM ideal for 3D intracellular imaging. The calculated anisotropy error in each pixel increases at the edges of the microspheres, a consequence of low count rates [26] , resulting in some noise artefacts and loss of anisotropy ( Supplementary Figs 6 and 7 ). However, anisotropy remained constant above a threshold that is determined by acquisition parameters and intrinsic noise ( Supplementary Fig. 6 ). Next we exploited the excellent optical sectioning properties for tomographic MFAM imaging of an optical phantom simulating a bound/unbound 3D environment. Two highly homogeneous populations of green-fluorescent microspheres with distinct anisotropy values ( Supplementary Figs 8 and 9 ) were suspended in a 2% agarose solution ( Fig. 3b ). In both the 3D FA colour-coded reconstructions and the optically sectioned planes, the two populations of microspheres are distinguishable throughout the entire phantom depth (ca. 90 μm) and assigned the correct anisotropy-based colour ( Fig. 3b and Supplementary Fig. 8b ). 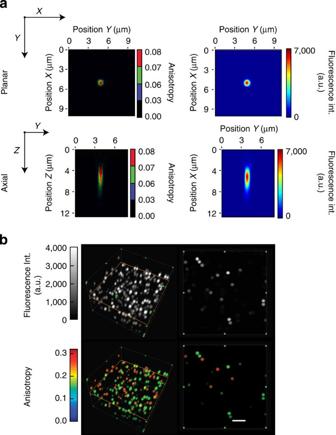Figure 3: Optical characterization of MFAM. (a) MFAM point spread function characterization. Planar and axial microscope FA and plain fluorescence images of a fluorescent microsphere. (b) 3D reconstructions of a mixture of two fluorescent microspheres populations with high and low anisotropy suspended in agarose, with the respective planar images obtained across the transversal plane indicated by the orange line. Anisotropy images colour-coded based on anisotropy values. Right: planar images across the transversal plane indicated (orange line). Top, fluorescence. Bottom, anisotropy. Scale bar, 20 μm. Figure 3: Optical characterization of MFAM. ( a ) MFAM point spread function characterization. Planar and axial microscope FA and plain fluorescence images of a fluorescent microsphere. ( b ) 3D reconstructions of a mixture of two fluorescent microspheres populations with high and low anisotropy suspended in agarose, with the respective planar images obtained across the transversal plane indicated by the orange line. Anisotropy images colour-coded based on anisotropy values. Right: planar images across the transversal plane indicated (orange line). Top, fluorescence. Bottom, anisotropy. Scale bar, 20 μm. Full size image Imaging drug–target engagement in live cells FA has traditionally been used to measure binding of small fluorescent molecules to a larger target biomolecule [27] . When bound, the increased molecular mass of the probe–target complex will result in a higher rotation correlation time τ θ limiting molecule rotation and increasing FA ( Fig. 4a ), while a shift in fluorescence lifetime could also change FA. Depending on its state (bound/unbound) a single fluorescent molecule can produce two values of anisotropy, and, because anisotropy is an additive property, the measured pixel value in an FA image is the fraction-weighted sum of the two possible anisotropy values within a voxel. MFAM measurements of Me 5 –BODIPY labelled Biotin (Biotin–BODIPY) indeed show an increase in anisotropy as a function of binding to NeutrAvidin ( Fig. 4a ) with a similar trend to single-photon measurements ( Supplementary Fig. 3 ), due to a change in τ θ ( Supplementary Methods ). 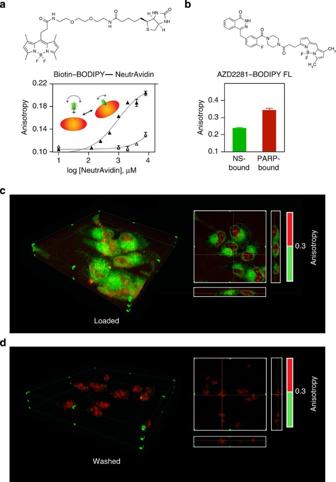Figure 4: Live cell imaging of target engagement. (a) The anisotropy value of Biotin–BODIPY (MW 676.62) increases as a function of binding to NeutrAvidin (MW 60 kDa) (filled triangles), which is suppressed in the presence of 10 × unlabelled biotin as competitor (open triangles). Shown are average±s.d. (n=3); curve fits added for trend visualization. Inset illustration: comparison between the rotation of a free fluorophore in solution and a fluorophore bound to a protein. Owing to the large difference in size of the ligand and the receptor, the increase in FA following binding is large. (b) Average±s.d. anisotropy of non-specifically interacting (green) and PARP bound (red) AZD2281–BODIPY FL (n=3). (c) 3D anisotropy image and corresponding planar and axial cross sections of live HT1080 cells loaded with AZD2281–BODIPY FL. Green corresponds to fluorescent drug molecules that are non-specifically bound. Red corresponds to fluorescent drug molecules with high anisotropy suggesting target (PARP) binding. Normal fluorescence images are shown inSupplementary Fig. 18. Scale bar, 16 μm. (d) 3D anisotropy image and corresponding planar and axial cross sections of live HT1080 cells loaded with AZD2281–BODIPY FL and washed for 30 min. Scale bars, 20 μm. Figure 4: Live cell imaging of target engagement. ( a ) The anisotropy value of Biotin–BODIPY (MW 676.62) increases as a function of binding to NeutrAvidin (MW 60 kDa) (filled triangles), which is suppressed in the presence of 10 × unlabelled biotin as competitor (open triangles). Shown are average±s.d. ( n =3); curve fits added for trend visualization. Inset illustration: comparison between the rotation of a free fluorophore in solution and a fluorophore bound to a protein. Owing to the large difference in size of the ligand and the receptor, the increase in FA following binding is large. ( b ) Average±s.d. anisotropy of non-specifically interacting (green) and PARP bound (red) AZD2281–BODIPY FL ( n =3). ( c ) 3D anisotropy image and corresponding planar and axial cross sections of live HT1080 cells loaded with AZD2281–BODIPY FL. Green corresponds to fluorescent drug molecules that are non-specifically bound. Red corresponds to fluorescent drug molecules with high anisotropy suggesting target (PARP) binding. Normal fluorescence images are shown in Supplementary Fig. 18 . Scale bar, 16 μm. ( d ) 3D anisotropy image and corresponding planar and axial cross sections of live HT1080 cells loaded with AZD2281–BODIPY FL and washed for 30 min. Scale bars, 20 μm. Full size image While dyes presenting longer lifetimes could be considered as alternative candidates, BODIPY was chosen due to unique characteristics that allow intracellular imaging. Specifically, (i) BODIPY is relatively non-polar with the chromophore presenting electrical neutrality, therefore minimizing perturbation to the modified drug; (ii) the relatively long lifetime (the BODIPY we use here has a measured lifetime ~4.0 ns) makes it particularly suitable for fluorescence polarization-based assay; (iii) BODIPY is highly permeant to live cells, easily passing through the plasma membrane, where it accumulates over time; (iv) it has a high extinction coefficient (EC >80,000 cm −1 M −1 ) and a high fluorescence quantum yield (often approaching 1.0, even in water); (v) it presents a lack of ionic charge and spectra that are relatively insensitive to solvent polarity and pH; and, (vi) finally, it has a large two-photon cross section. Although most BODIPY dyes enjoy a relatively long lifetime, dyes such as Cy3 and the Alexa dyes will be inefficient for FA imaging, with their lifetimes so short that the anisotropy of the unbound probe will be near the fundamental anisotropy, and hence indistinguishable from the bound probe. Conversely, fluorophores with extremely long lifetimes, or phosphorescence emission, are also unsuitable as the increase in rotation correlation time will not be large enough to increase the anisotropy. It is therefore important to characterize the lifetime, by fluorescence lifetime imaging microscopy (FLIM), of the possible candidate dyes for drug labelling that could be potentially used for two-photon fluorescence polarization imaging. Also, dyes presenting changes in their quantum yield upon binding will bias the readout value of total anisotropy affecting the measured binding isotherm. To test the MFAM imaging approach in a relevant drug–target system, we chose to target poly(ADP-ribose) polymerase (PARP) with the small-molecule inhibitor Olaparib (AZD2281) that had been modified to bear a BODIPY-FL handle [7] . This model system and its cellular location had previously been well validated [7] , [28] . PARP comprises a family of enzymes that are required for DNA repair [29] , [30] , [31] , and therefore present a potential chemotherapeutic target through inhibition. Owing to the high molecular weight of PARP1 (~120 kDa) a significant increase in anisotropy is observed for ‘target-bound’ over ‘free’ or ‘intracellular drug’ AZD2281–BODIPY FL, respectively ( Fig. 4b and Supplementary Fig. 10a ). An anisotropy threshold can then be assigned to distinguish between the bound states and MFAM intracellular imaging of drug–target engagement can be obtained in 3D ( Fig. 4c,d : red, PARP bound; green, ‘intracellular drug’). When incubated with AZD2281–BODIPY FL we observed rapid accumulation throughout the entirety of each HT1080 cell. Intracellular drug was present in the cytoplasmic region, while bound drug was present in the nucleus ( Fig. 4c and Supplementary Fig. 11 ), which colocalized with PARP immunostaining [28] ( Supplementary Fig. 10b ). Following extended washing cycles, the cytoplasmic AZD2281–BODIPY FL is cleared, while the nuclear, bound drug remains ( Fig. 4d ). Similar nuclear binding of AZD2281–BODIPY FL was observed in other cell lines reported to express PARP as well ( Supplementary Fig. 12 ), as validated previously [28] . Real-time in vitro measurements ( Fig. 5 ) show AZD2281–BODIPY FL accumulated in the cytoplasm significantly more than in the nucleus, which is likely the result of interactions with intracellular membranes. Yet, only the nucleus presents high values of anisotropy, suggesting PARP binding ( Fig. 5a ). The high nuclear anisotropy ( Fig. 5a ) is not observed in the presence of unlabelled AZD2281 as competitor (5 × ) ( Fig. 5b ), which further suggests the high anisotropy measured in the nuclei was due to drug–target binding and not induced by potential artefacts, such as viscosity. In addition, there was no target binding of AZD2281–BODIPY FL in the cytoplasm, as demonstrated by the significant difference between nuclear and cytoplasmic anisotropy throughout the course of loading and washing as well as the insignificant difference between cytoplasmic anisotropy in the non-competitive and competitive experiments ( Fig. 6 ). Constant anisotropy with decreasing intensity in the cytoplasm in both non-competition and competition experiments indicates that homo-FRET was not the cause of the lower anisotropy ( Fig. 6 ). Additionally, high nuclear anisotropy is not caused by the BODIPY FL itself ( Supplementary Fig. 13 ). Finally, there was no significant difference in fluorescence lifetime between nuclear and cytoplasmic regions in loaded HT1080 cells ( Supplementary Fig. 14 ). Through washing and competition experiments, bound and unbound values of anisotropy in the nucleus can be determined, and the percentage of target-bound AZD2281-BODIPY FL can be calculated at any point in time ( Supplementary Fig. 15 ). 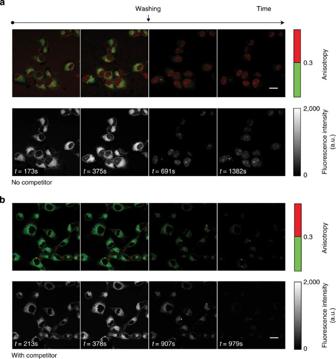Figure 5: Imaging target engagement over time. (a) Anisotropy and corresponding fluorescence images of AZD2281–BODIPY FL at four representative time points during drug loading and after washing. (b) Similar experiment as in (a) but in the presence of fivefold higher concentration of unlabelled AZD2281 (competition). Scale bars, 20 μm. Figure 5: Imaging target engagement over time. ( a ) Anisotropy and corresponding fluorescence images of AZD2281–BODIPY FL at four representative time points during drug loading and after washing. ( b ) Similar experiment as in ( a ) but in the presence of fivefold higher concentration of unlabelled AZD2281 (competition). Scale bars, 20 μm. 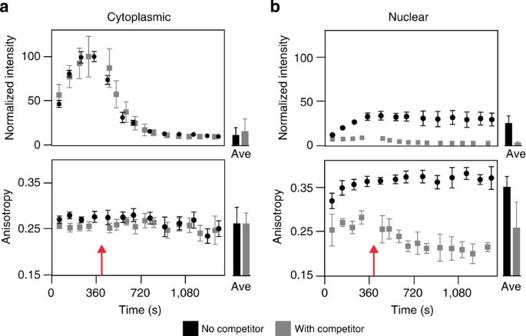Figure 6: Real-time imaging of drug–target engagement in live cells. Normalized intensity and anisotropy as a function of time for HT1080 cells loaded with AZD2281–BODIPY FL and washed. Values are measured in both the cytoplasmic (a) and nuclear (b) regions of the cells in the absence (black circles) and presence (grey squares) of fivefold higher concentration of unlabelled AZD2281 (competition). Points in the graphs refer to a single experiment, average±s.d. (n=6 cells). Also shown at the right of each figure, average±s.d. at the end of the wash in the absence (black bars,n=42 cells, seven separate experiments) and presence (grey bars,n=36 cells, six separate experiments) of unlabelled AZD2281 (5 × ). Bars are representative of seven and six different experiments, respectively. Red arrows indicate switch from loading to washing. Fluorescence intensity refers to the sum of both perpendicular and parallel channels. Full size image Figure 6: Real-time imaging of drug–target engagement in live cells. Normalized intensity and anisotropy as a function of time for HT1080 cells loaded with AZD2281–BODIPY FL and washed. Values are measured in both the cytoplasmic ( a ) and nuclear ( b ) regions of the cells in the absence (black circles) and presence (grey squares) of fivefold higher concentration of unlabelled AZD2281 (competition). Points in the graphs refer to a single experiment, average±s.d. ( n =6 cells). Also shown at the right of each figure, average±s.d. at the end of the wash in the absence (black bars, n =42 cells, seven separate experiments) and presence (grey bars, n =36 cells, six separate experiments) of unlabelled AZD2281 (5 × ). Bars are representative of seven and six different experiments, respectively. Red arrows indicate switch from loading to washing. Fluorescence intensity refers to the sum of both perpendicular and parallel channels. Full size image In vivo imaging of drug–target engagement Finally, we used MFAM for in vivo imaging applications. In biological diffusive samples multiple scattering events limit the imaging depth by reducing the number of excitation photons in the focal area while decreasing the number of collected photons [32] . A decrease of the degree of polarization with resulting lower values of anisotropy is therefore present as evidenced on tissue phantom measurements ( Supplementary Fig. 16 , Supplementary Methods ). To better characterize how diffusion and absorption limit the effective anisotropy imaging depth we first injected fluorescent microspheres into superficial tissue within a nude mouse dorsal window chamber ( Fig. 7a ). In vivo MFAM measurements indicated a slight depth-dependent loss of anisotropy ( Fig. 7b ), with a 10% loss at 100 μm, which, based on the anisotropy difference in binding measurements, does not affect target engagement measurements. 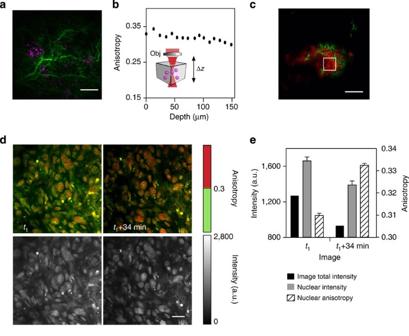Figure 7: Imaging of AZD2281–BODIPY FL target engagement in a live mouse. (a)In vivofluorescence image of injected fluorescent microspheres (pink) in the vascularized (green) tissue fascia of a mouse DSC. Scale bar, 50 μm. (b) Anisotropy of the injected fluorescent microspheres as a function of depth within the tissue fascia. Each point corresponds to a single bead measurement. (c) Confocal fluorescence image of HT1080 H2B mApple cells (red) in a mouse DSC. After 1–2 weeks, the tumour area is highly vascularized and, upon intravenous injection, perfused with AZD2281–BODIPY FL (green). The white square indicates the imaged area in (d). Scale bar, 100 μm. (d)In vivoanisotropy (top) and fluorescence (bottom) images of AZD2281–BODIPY FL following intravenous infusion (left) and 34 min later (right). Scale bar, 20 μm (e) Overall image intensity (black), nuclear intensity (grey) and nuclear anisotropy (unfilled, striped) as measured from the images in (d). Nuclear intensity and anisotropy values are average±s.e. (n=90 for imaget1,n=102 for imaget1+34 min). Fluorescence intensity refers to the sum of both perpendicular and parallel channels. Figure 7: Imaging of AZD2281–BODIPY FL target engagement in a live mouse. ( a ) In vivo fluorescence image of injected fluorescent microspheres (pink) in the vascularized (green) tissue fascia of a mouse DSC. Scale bar, 50 μm. ( b ) Anisotropy of the injected fluorescent microspheres as a function of depth within the tissue fascia. Each point corresponds to a single bead measurement. ( c ) Confocal fluorescence image of HT1080 H2B mApple cells (red) in a mouse DSC. After 1–2 weeks, the tumour area is highly vascularized and, upon intravenous injection, perfused with AZD2281–BODIPY FL (green). The white square indicates the imaged area in ( d ). Scale bar, 100 μm. ( d ) In vivo anisotropy (top) and fluorescence (bottom) images of AZD2281–BODIPY FL following intravenous infusion (left) and 34 min later (right). Scale bar, 20 μm ( e ) Overall image intensity (black), nuclear intensity (grey) and nuclear anisotropy (unfilled, striped) as measured from the images in ( d ). Nuclear intensity and anisotropy values are average±s.e. ( n =90 for image t 1 , n =102 for image t 1 +34 min). Fluorescence intensity refers to the sum of both perpendicular and parallel channels. Full size image After determining that our technique is viable in an in vivo setting we measured drug–target engagement in a mouse. Intravenous delivery to an implanted HT1080 cell tumour showed AZD2281–BODIPY FL diffusion into the cancer cells ( Fig. 7c ). Cells expressing nuclear mApple-labelled H2B, which did not affect AZD2281 anisotropy measurements ( Supplementary Figs 11 and 17 ), were used to locate the tumour [33] . Binding of AZD2281–BODIPY FL to PARP in the nucleus occurred immediately upon drug infusion ( Fig. 7d ). The bound fraction of the drug was retained in the nucleus while the unbound extracellular and cytoplasmic drug was cleared away over time ( Fig. 7d ). Both the nuclear and overall fluorescence intensity decreased over time; however, the nuclear anisotropy increased as unbound AZD2281–BODIPY FL was cleared ( Fig. 7e ). The ability to measure the pharmacology of drugs on a molecular level in live cells represents one of the greatest challenges in chemical biology and drug discovery [9] . Currently, there are no demonstrated methods for direct measurements. Subsequently, all information is based on indirect or artificial approaches that do not provide the spatiotemporal resolution and accuracy required to establish reliable models and/or do not occur in biologically relevant settings. Here we have developed a promising novel approach utilizing MFAM, which, for the first time, allows direct visualization of target-bound versus unbound small-molecule drugs in real time. Using a chemotherapeutic compound in Phase III clinical trials, we demonstrate that our approach is not only applicable to live cultured cells but also enables real-time imaging of drug–target engagement in vivo and with submicron resolution. Our technique does not require separation between bound and free compound, is not limited to equilibrium analysis and does not affect the biological settings. As such, MFAM offers a new and fundamental imaging platform for accelerating translational drug development through insight into in vivo drug activity and inefficacy. Cell culture HT1080 cells (ATCC) stably expressing H2B mApple fluorescent protein [28] , [33] , [34] were cultured in DMEM with 10% FBS, 1% pen-strep and 100 μg ml −1 geneticin (Invitrogen). HT1080 cells were cultured in DMEM with 10% FBS and 1% pen-strep. MDA-MB-436, HCC1937 and MHH-ES1 cells were cultured in RPMI with 10% FBS and 1% pen-strep. Cells were plated onto 25 mm no. 1 cover glass for in vitro imaging. Tumour model All animal experiments were performed in accordance with the Institutional Animal Care and Use Committee at Massachusetts General Hospital. Female 20-week-old nude mice (Cox-7, Massachusetts General Hospital, Boston, MA, USA) were used. All surgical procedures were conducted under sterile conditions and facilitated through the use of a zoom stereomicroscope (Olympus SZ61). During all surgical procedures and imaging experiments mice were anaesthetized by isofluorane vaporization (Harvard Apparatus) at a flow rate of 2 l per min of isofluorane: 2 l per mine of oxygen. The body temperature of the mice was kept constant at 37 °C during all imaging experiments and surgical procedures. Dorsal skinfold window chambers (DSC) were implanted 1 day before imaging following a well-established protocol. Briefly, the two layers of skin on the back of the mouse were stretched and kept in place by the DSC. One skin layer was surgically removed and replaced by a 12-mm diameter glass cover slip positioned on one side of the DSC, allowing for convenient access and imaging of the tumour area. A spacer located on the DSC prevented excessive compression of both tissue and vessel, guaranteeing good vascular perfusion within the tumour region. HT1080 H2B mApple cells were harvested by trypsinization (0.25% trypsin:EDTA) and resuspended in PBS. Mice were anaesthetized and ~10 6 cells (100 μl 1 × PBS) were injected subcutaneously into the back of female Nu/Nu mice (Cox-7, Massachusetts General Hospital) aged 20–25 weeks in a 1:1 mixture of Matrigel (BD Biosciences). Cells were injected using a 0.5-ml insulin syringe with the needle bent at 90 degrees to better control the position of the injection site. In order to allow for the tumour to be established and neovascularization to occur, the tumours were allowed to grow for 1–2 weeks before DSC implantation. Microscope configuration The optical set-up is based on a custom-modified Olympus FV1000-MPE (Olympus, USA) laser scanning microscopy system equipped with an upright BX61-WI microscope (Olympus, USA) and is illustrated in details in Fig. 1b . Excitation light (red beam) from a Ti:sapphire laser (L) is filtered to select a linear state of polarization and then focused onto the imaged sample. Emitted fluorescent light (green beam) is epi-collected, separated into two linearly polarized orthogonal components and spectrally filtered before non-descanned detection. The MaiTai DeepSee Ti:sapphire pulsed laser (Spectra Physics) had a pulse-width of 110 fs and a repetition rate of 80 MHz. Laser was tuned at 910 nm for two-photon excitation of Me 5 –BODIPY and BODIPY FL. A Glan–Thompson polarizer (Newport) and a half-wave plate (Thor Labs) were inserted in the laser path toward the objective in order to create a linear state of polarization aligned along a fixed predetermined axis. Light was then focused onto the sample with a × 25 1.05 NA water-immersion objective (XLPlan N, 2 mm working distance, Olympus). Fluorescence emission was detected in epi-collection mode through the same focusing objective. A dichroic filter (690 nm) diverted the fluorescent light towards a non-descanned detection path, followed by a low-pass filter (685 nm). Along the detection path a polarizing beam splitter (Edmund optics) was inserted to separate the light in two orthogonal states of polarization, each one followed by a band-pass filter (490–540 nm, Chroma). Orthogonal and parallel linear polarized light was then focused and detected by two separate photomultiplier tubes ( I || , I ⊥ ). The excitation light was linearly polarized to be parallel and perpendicular aligned to the two PMTs. Dual detector acquisition is recommended to avoid severe anisotropy artefacts induced by intensity fluctuations. The imaging system was also operated in confocal modality. Me 5 –BODIPY (Exc: 493 nm; Em: 503 nm), BODIPY-FL (Exc: 503 nm, Em: 512 nm), Fluorescein (Exc: 494 nm, Em: 521) and H2B mApple (Exc: 568 nm, Em: 592 nm) were scanned and excited sequentially using a 473 and a 559-nm diode laser, respectively, in combination with a DM488/559-nm dichroic beam splitter. Emitted light was then separated and collected using an SDM560 beam splitter and BA490-540 and BA575-675 band-pass filters (Olympus, USA). Confocal large field-of-view images were acquired using a × 2 air objective (XL Fluor 2x/340 NA 0.14) and a water-immersion objective with a high numerical aperture (NA) and large working distance (XLPlan N × 25, NA 1.05, w.d. 2 mm, Olympus) were utilized. 3D multichannel serial imaging was obtained through the use of a built-in Z axis motor with a 0.01 μm step size. Different areas along the entire size of the dorsal window chamber were sequentially imaged over time using a microscope-controlled long-range XY axis translation stage. Optical characterization of the system All polarizer, optical filters, polarization beam splitter, half-wave plate and Glan–Thompson polarizer were tested and characterized. Light from the laser was first linearly polarized using a Glan–Thompson polarizer and then aligned along a defined arbitrary axis with the use of a half wave plate. Light at the entry of the objective was measured using a polarizer and a photodetector to confirm the state of polarization remained linear along its path to the objective. Photodetectors were tested for any polarization dependence. The path from the objective to the photodetectors was also tested to assure that equal distribution of power is present between the two detectors. Voltage of the two photodiodes was slightly adjusted in order to fine-tune equal signal detection. The noise contribution of the two detectors was equal for all in vitro and in vivo measurement conditions. The two detectors responded with the same linear curve along the measurement range. Calibration of the MFAM systems was performed using a set of angle-adjustable linear polarizer placed in front of the detectors, and at the entry of the objective. Fluorescein in water at room temperature was used to fine-tune the voltage gains on the two individual PMT sensors. The solution (5 μl) was placed between a microscope slide and a cover glass and imaged. Settings were regulated such that 2 μM fluorescein solution produced an anisotropy of 0.004 after correction of the G factor. The gains settings were then maintained throughout the entirety of all measurements. To check reproducibility over days, fluorescence slides containing uniformly distributed fluorophores were measured before each imaging session. Images of three different slides (each one with a different fluorophore) were taken during each imaging session to confirm that the measured anisotropy during the session matched the previous measurements. Images of the slides were taken over various time periods and at varying excitation intensity for system characterization. Thermal variation can cause slight difference on a day-to-day basis. To compensate for them the microscope is located within a thermally stable isolating cage, mounted on an aluminium frame. Measurements over time within the same day and over several days indicate strong reproducibility in FA measurements ( Supplementary Fig. 19 ). Polarization distortions due to dichroic beam splitter reflections and the objective’s high numerical aperture [35] , such is the requirement for multiphoton microscopy, can lead to anisotropy artefacts in particular when imaging over the entire objective field of view [36] . While compensation could be used through different calibration methods, images collected over a restricted field of view eliminate any edge artefact ( Supplementary Figs 4 and 5 , Supplementary Methods ). Me 5 –BODIPY was brought up in DMSO (Sigma) to a 1 mM stock solution. Solutions of a final concentration of 20 μM Me 5 –BODIPY in DMSO were mixed with glycerol (Sigma) to create varying concentrations of glycerol. Images of 5 μl drops of solution inserted between the cover glass were taken at each glycerol concentration in triplicate. 3D anisotropy phantom Six-micrometre green-fluorescent microspheres (InSpeck Microscope Image Intensity Calibration Kits, Invitrogen) were used for demonstrating optical sectioning capabilities. Each kit consists of seven different types of microspheres with fluorescence intensities ranging from very low to very bright (100%, 30%, 10%, 3%, 1%, 0.3% and non-fluorescent). The fluorescence intensity of the microspheres within each vial is defined with respect to that of the microspheres with the highest fluorescence (that is, 100%). We selected one vial containing the brightest microspheres (that is, 100%) and another vial containing the next brightest (30%) microspheres. The fluorescence intensity of the microspheres in each vial is highly homogeneous, as shown in Supplementary Fig. 8 . Importantly, their value of anisotropy is not dictated by the lifetime ( Supplementary Fig. 9 ) or mobility of dye within the microspheres, but instead by a concentration-dependent effect (homo-FRET) (see ref. 26 for a detailed explanation of the effect). Owing to homo-FRET, the two populations of microspheres present different values of anisotropy with a highly homogenous distribution (0.274±0.008 and 0.193±0.005; Supplementary Fig. 8 ). The microspheres are therefore useful for testing anisotropy distributions in phantoms [26] . The two populations of microspheres were mixed in equal proportion, suspended in 2% agarose and allowed to solidify between two pieces of cover glass before imaging. Point spread function measurements One-micrometre green fluorescence microspheres (Bangs Labs) on cover glass were also imaged and used for point spread function characterization. Tissue phantoms The tissue optical phantoms used for characterization ( Supplementary Methods ) contained fluorescein (20 μM) (Sigma), which was diluted in 1% Intralipid (10% Solution, Baxter Healthcare) in PBS with varying concentrations of India ink following a well-established protocol [37] . The corresponding scattering coefficient μ ′ s was equal to 11 cm −1 , a value typically considered for mouse tissue phantoms [37] . Optical densities of ink concentrations in PBS were determined by measuring the absorbance spectrum at 910 nm. Fluorescent images of the solution were taken at 10-μm intervals through the depth of the phantoms. FLIM measurements Fluorescence lifetime imaging was performed using a Zeiss 710 confocal NLO laser scanning system on an upright Zeiss Examiner stand with a × 40 NA 1.1 water-immersion LD C-Apochromat objective and a Becker & Hickl TCSPC system. Two-photon excitation was achieved using a Coherent Chameleon Vision II tunable laser (680–1,040 nm) that provided 140-fs pulses at a 80-Mhz repetition rate with an output power of 3 W at the peak of the tuning curve (800 nm). Laser scanning was controlled by Zeiss Zen software and set to a pixel dwell time of 1.58 μs and 0.9-s frame rate at 910 nm wavelength excitation. Enhanced detection of the scattered component of the emitted (fluorescence) photons was afforded by the use of a Becker & Hickl HPM-100-40 hybrid detector, which incorporates the Hamamatsu R10467 hybrid PMT tube. Imaging was performed in the dark with blackout enclosure around the microscope to exclude external sources of light during the sensitive period of FLIM measurement. Emitted fluorescence was deflected to the non-descanned light path via a 760+ mirror and emission range was limited to 500–550 nm by a Chroma filter in front of the HPM-100-40 detector. Acquisition time was typically 60 s with a count rate of 2–5 × 10 4 photons per second. Photon counting and electronic timing synchronization was controlled and measured with a Becker & Hickl TCSPC electronics (SPC-830) and SPCM software (Becker & Hickl GmbH) Lifetime decay of the fluorescence was analysed with SPCImage software (Becker & Hickl GmbH). Plate reader anisotropy measurements Single-photon data were collected in a plate reader set up for fluorescence polarization measurements (Tecan Sapphire 2). A G-factor for the instrument was calculated from 2 μM fluorescein in water. Measurements were performed in 96- or 384-well plates. Biotin–BODIPY FL and NeutrAvidin binding Biotin was conjugated to Me 5 –BODIPY (Biotin–BODIPY) and brought to 1 mM stock solution in DMSO. Biotin–BODIPY (10 μM) was mixed with varying concentrations of NeutrAvidin (Thermo Scientific) in PBS with 1% Triton X (Sigma). Each sample was imaged in triplicate as a drop between a microscope slide and cover glass. Measurements of each sample were also performed using single-photon excitation in a plate reader. Measurements were also made in the presence of 100 μM free Biotin to competitively compete with the Biotin–BODIPY. Free-molecule anisotropy AZD2281 labelled with BODIPY FL (AZD2281–BODIPY FL) was prepared as previously described [7] , [38] . PARP1 (BioVision) was brought up in the manufacturer’s recommended solution and added at 1.6 × the concentration of AZD2281–BODIPY FL (5 μM) in imaging media containing 2.5% FBS. Free AZD2281–BODIPY FL (5 μM) (no PARP) in the same imaging media with 2.5% FBS and in DMSO solutions were also prepared. Images were taken of drops of solution between cover glass. In vitro cellular imaging Cells on 25 mm cover glass were mounted into a closed bath perfusion chamber (Warner Instruments) and perfused with a custom perfusion system that enabled solution switching in the imaging chamber. Cells were imaged in phenol red-free DMEM with 10% FBS and 1% pen-strep. AZD2281–BODIPY FL (1 μM) was perfused into the imaging chamber followed by a washout with drug-free media. Images were obtained during the entire time interval at regular time points. For competition experiments, free AZD2281 (5 μM) (Selleck Chemicals) was added to the incubating solution before, during and after AZD2281–BODIPY FL addition. Me 5 –BODIPY was used for fluorophore control experiments. In vivo imaging Mice were anaesthetixed as indicated above. When imaged for prolonged period of time, the isoflurane flow rate was reduced to ~1 l per min. The DSC was inserted onto a custom stabilization plate to prevent image motion artefacts and axial drifts over the time of the imaging session. Plane tracking to ensure that the same area is imaged repeatedly over the course of the drug uptake measurements was achieved through the use of a built-in Z axis motor. Animals were warmed with a heating plate in order to keep their temperature constant. Green-fluorescent microspheres (2.5 μm; (InSpeck, Invitrogen) were dried out using an EZ-2 evaporator (Genevac) and resuspended in sterile PBS. After sonication, the microspheres were then injected into the skin tissue of a dorsal window chamber on a nude mouse. Injections were performed with a CellTram vario (Molecular Devices) through pulled glass pipettes. After the skin tissue absorbed the PBS, images of the microspheres were taken at increasing depths. The vasculature in the window chamber was imaged under bright-field with a CCD camera using a × 2 objective and overlaid with a fluorescence image using the same objective. AZD2281–BODIPY FL (7.5 μl in DMSO) was mixed with 30 μl of 1:1 solutol:dimethylacetamide (Sigma) and slowly added to 112.5 μl of PBS. The drug was injected through a tail vein intravenously and imaged with MFAM using a × 25 objective. Confocal images of drug infusion into the tumour were taken using a × 2 objective. Image processing During image acquisition in two-photon microscopy only a small number of photons are typically measured by the photodetectors with numbers ranging from tens to a few thousands with a statistical variation in the recorded number following a Poisson model of the noise. At lower counts per pixel, the error on the calculated anisotropy value will be then increasingly higher, giving rise to images presenting severe noise artefacts (a rigorous treatment on the role of photon statistics on fluorescence polarization can be found in ref. 26 ). To account for noise-induced variation we decided therefore to statistically weight every pixel anisotropy value within each image by its corresponding total intensity. Intensity-weighted images were created by assigning colours based on anisotropy values, indicated by the scale bar, to each pixel in the fluorescence image. The intensity of the image is therefore dependent on the fluorescence intensity, while the colour is dependent on the calculated anisotropy. In addition a BM3D collaborative filter was applied on each image [39] . Data analysis Images were analysed in Matlab (Mathworks) and ImageJ. All anisotropy measurements were calculated from the equation r =( I || − I ⊥ )/( I || +2 I ⊥ ). The detector noise of the two photodetectors was subtracted from the whole images before the data were processed. Fluorescence intensity refers to the sum of both perpendicular and parallel channels. Anisotropy values were obtained by defining a region of interest and measuring the average anisotropy within that region. Regions were extended to fluorescent images to calculate the corresponding intensity. How to cite this article: Dubach, J. M. et al. In vivo imaging of specific drug–target binding at subcellular resolution. Nat. Commun. 5:3946 doi: 10.1038/ncomms4946 (2014).